Origins of hydration lubrication Why is friction in healthy hips and knees so low? Hydration lubrication, according to which hydration shells surrounding charges act as lubricating elements in boundary layers (including those coating cartilage in joints), has been invoked to account for the extremely low sliding friction between surfaces in aqueous media, but not well understood. Here we report the direct determination of energy dissipation within such sheared hydration shells. By trapping hydrated ions in a 0.4–1 nm gap between atomically smooth charged surfaces as they slide past each other, we are able to separate the dissipation modes of the friction and, in particular, identify the viscous losses in the subnanometre hydration shells. Our results shed light on the origins of hydration lubrication, with potential implications both for aqueous boundary lubricants and for biolubrication. Friction between sliding surfaces in living systems is often at levels that engineers can only envy. Thus, friction coefficients of order 10 −3 , at pressures exceeding 100 atm, typical of articulating cartilage surfaces in healthy human joints [1] , cannot be reproduced by any synthetic surfaces, and its molecular-level understanding remains elusive [2] . Over the past decade, the concept of hydration lubrication has been invoked to account for the extremely low sliding friction observed at high pressures between charged surfaces in high-salt solution [3] , [4] , [5] , or when coated by surfactants [6] , [7] , [8] , liposomes [9] or hydrated polymer brushes [10] , [11] , [12] —boundary layers resembling those at articular cartilage surfaces [12] , [13] . According to this, hydration shells formed by water molecules are tenaciously attached to the charges they surround, and so cannot be easily squeezed out on compression [14] , [15] , [16] , [17] , [18] , yet are labile and so respond to shear in a fluid manner. However, there is little microscopic understanding of this mechanism, especially of the frictional dissipation within the subnanometre hydration shells that form its basic elements. This is because in all relevant studies to date, including refs 4 , 5 , 6 , 7 , 8 , 9 , 10 , 11 , the measured friction may have been dominated by other dissipation pathways, such as polymer chains disentangling past each other [10] , [11] or distortion of sheared liposomes [9] . The present study overcomes these limitations by trapping hydrated ions in the gap between molecularly smooth surfaces, and measuring the friction between them as they slide at pressures and shear rates one to two orders of magnitude higher than previously achieved [3] . This allows a clear separation of different dissipation regimes, and enables to isolate the dissipation arising from shear of the subnanometre hydration shells themselves, which are intrinsic to all hydration lubrication processes, from any system-dependent dissipation. Our results reveal that viscous dissipation within hydration shells—for the ions examined—is some 250-fold larger than the viscosity either of bulk water or of similarly confined non-hydration water. This sheds strong light on the origins of hydration lubrication, with implications both for aqueous boundary lubricants and for lubrication in biological systems. Normal surface forces We use a surface force balance (SFB) with state-of-the-art resolution and sensitivity in measuring interactions, particularly shear forces, between curved, atomically smooth mica surfaces (mean radius of curvature R ≈1 cm), across nanometre and subnanometre liquid films, as described in detail earlier [3] (Methods) and schematically shown in the inset of Fig. 1 . Here we measure the normal and shear forces, F n ( D ) and F s ( D ), respectively, between such surfaces at separation D , across highly pure aqueous solutions of ca 0.1 M NaNO 3 or NaCl at mean pressures P and sliding velocities ν s that are up to two orders of magnitude higher than in earlier studies [3] , [19] (Methods). 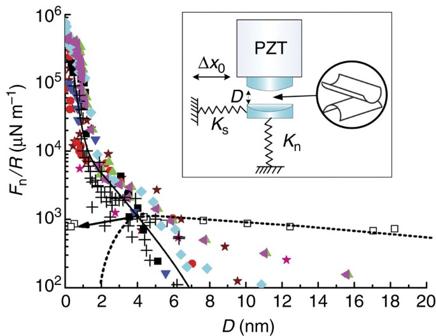Figure 1: Normal forces across confined hydrated ions. Profile of normal forcesFn(D) versus surface separationDbetween curved mica surfaces (mean radius of curvatureR≈1 cm, see schematic inset), across 0.1 M sodium salt solutions (both NaCl and NaNO3: there is no systematic difference between them). Data are for both first and subsequent approaches at a given point following shear measurements, indicating absence of any surface damage up to the highest loads. Different symbols (coloured to highlight difference) correspond to different contact points, including different experiments. Also shown (empty squares) is the control pure water profile (no added salt), with arrow indicating jump into adhesive contact. The profiles are normalized asFn(D)/RversusDto yield the interaction energy per unit area between flat parallel plates obeying the same force law in the Derjaguin approximation (within a factor 2π). The solid lines are a fit to a Derjaguin–Landau–Vervey–Overbeek expression (DLVO), together with a short-ranged exponential term (inEh,Dh) representing the hydration forces15:Fn/2πR=64ckBTκ−1tanh2(eψ0//kBT) exp (−κD)–AH/12πD2+Ehexp(−D/Dh), wherecis the electrolyte concentration in mol dm−3,Tis the temperature (296±1 K),kBis Boltzmann’s constant,AHis the Hamaker constant of mica across water (2 × 10−20J) andψ0andκ−1are, respectively, the effective (large-separation) surface potential and the Debye length. The fit values areψ0=70 mV,κ−1=1.36 nm,Eh=0.23 J m−2andDh=0.2 nm. The cross-symbols are from previous studies for similar NaCl concentrations3,18. The dotted line for the pure water control is a fit to the DLVO expression withψ0=140 mV,κ−1=70 nm andAHas above, whereas the arrow shows the jump of the surfaces into adhesive contact, which also reveals directly the bulk-like viscosity of the confined pure water29before adding salt. The inset shows the schematic SFB configuration (Methods). Figure 1 shows the normalized force profiles F n ( D )/ R versus D across water (always taken as a control for system cleanliness before adding salt) and across the 0.1 M salt solutions, revealing the longer-ranged repulsion arising from counterion osmotic pressure [18] , [20] down to D ≈2 nm. At D <ca 2 nm, we observe the characteristic repulsion arising from the tightly bound hydration shells [14] , [15] , [16] , [17] , [18] surrounding the Na + counterions trapped between the negatively charged mica surfaces. Figure 1: Normal forces across confined hydrated ions. Profile of normal forces F n ( D ) versus surface separation D between curved mica surfaces (mean radius of curvature R ≈1 cm, see schematic inset), across 0.1 M sodium salt solutions (both NaCl and NaNO 3 : there is no systematic difference between them). Data are for both first and subsequent approaches at a given point following shear measurements, indicating absence of any surface damage up to the highest loads. Different symbols (coloured to highlight difference) correspond to different contact points, including different experiments. Also shown (empty squares) is the control pure water profile (no added salt), with arrow indicating jump into adhesive contact. The profiles are normalized as F n ( D )/ R versus D to yield the interaction energy per unit area between flat parallel plates obeying the same force law in the Derjaguin approximation (within a factor 2 π ). The solid lines are a fit to a Derjaguin–Landau–Vervey–Overbeek expression (DLVO), together with a short-ranged exponential term (in E h , D h ) representing the hydration forces [15] : F n /2 πR =64 c k B T κ −1 tanh 2 ( eψ 0/ /k B T) exp (− κD )–A H /12 πD 2 + E h exp(− D / D h ), where c is the electrolyte concentration in mol dm −3 , T is the temperature (296±1 K), k B is Boltzmann’s constant, A H is the Hamaker constant of mica across water (2 × 10 −20 J) and ψ 0 and κ −1 are, respectively, the effective (large-separation) surface potential and the Debye length. The fit values are ψ 0 =70 mV, κ −1 =1.36 nm, E h =0.23 J m −2 and D h =0.2 nm. The cross-symbols are from previous studies for similar NaCl concentrations [3] , [18] . The dotted line for the pure water control is a fit to the DLVO expression with ψ 0 =140 mV, κ −1 =70 nm and A H as above, whereas the arrow shows the jump of the surfaces into adhesive contact, which also reveals directly the bulk-like viscosity of the confined pure water [29] before adding salt. The inset shows the schematic SFB configuration (Methods). Full size image Shear forces across hydrated ions To elucidate the nature of the frictional dissipation, we measured the dependence of the shear forces F s on ν s at different P and corresponding surface separations D . By substantially increasing both P (which enabled us to work at D below 0.8 nm) and especially ν s in the present experiments, we were able to measure F s values significantly above the noise level (which limited earlier studies [3] , [19] , see later). Typical time traces of the shear forces are shown in Fig. 2 . 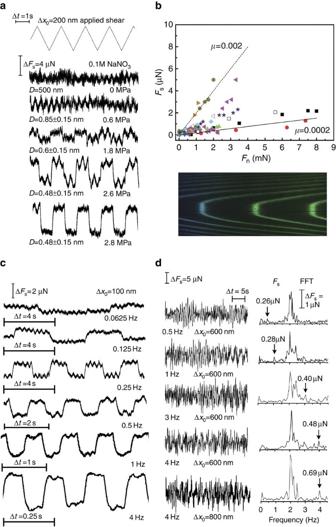Figure 2: Shear forces across confined hydrated ions. Sets of time (t) traces of shear forcesFs(t,P,νs) between mica surfaces across 0.1 M Na+salts, at different pressuresPand sliding velocitiesνs, taken directly from the SFB. Traces are monitored via bending of the shear springsKsin response to back-and-forth lateral motion Δx0applied to the top surface (for example, top trace ina), see inset toFig. 1. (a) Typical traces showing variation ofFswith increasing loadsFn, corresponding to increasingP, at fixedνs(200 nm s−1). Extraction of signals from noisy profiles is described below (d). In other measurements,Fswas determined at decreasingFnandP. (b) Summary ofFsversusFndata from traces such as ina, atνs=200 nm s−1. The lines correspond to friction coefficientsμ(=Fs/Fn) as indicated. Different symbols (coloured to highlight difference) correspond to different contact points, including different experiments. Full symbols: increasingFn; empty symbols: decreasingFn, and each shape of symbols is for increasing or decreasing load at a given contact point. The lower inset shows typical fringe-tip flattening at highP(enabling checks of the Hertzian expression used to evaluateP, Methods). (c,d) TypicalFs(t,νs) traces at the high (Fn=6 mN) and low (Fn=0.1 mN) load regimes, respectively, at fixed loadsFn, at increasing velocitiesνsapplied to the top surface. In other measurements,Fswas determined at decreasingνs. For the traces shown, the amplitudes Δx0indicated are fixed, whereas the frequencies vary as shown. Where the signal is comparable with the noise level, as inb, theFsvalues are extracted at the respective drive frequencies using Fast Fourier Transform of the data to frequency (ω)-dependentFs(ω), as indicated on the right ofd. Figure 2a shows F s at increasing load F n at a fixed ν s , with a summary of the F s versus F n variation given in Fig. 2b ; whereas Fig. 2c,d shows F s at increasing ν s at two load regimes (the high-load and the low-load regimes) differing by some two orders of magnitude. The top trace in Fig. 2a shows the back-and-forth motion of the upper confining mica surface, whereas the lower traces show the shear force transmitted to the lower surface across the confined film. The frequency dependence of F s , on the right of Fig. 2d , enables extraction of the shear force at the drive frequency from the noisy signal. We note that, within the scatter for a given contact point, the shear forces vary reversibly with the shear velocity and with normal load, indicating that no surface damage occurs during the shear (Methods). Figure 2: Shear forces across confined hydrated ions. Sets of time ( t ) traces of shear forces F s ( t , P , ν s ) between mica surfaces across 0.1 M Na + salts, at different pressures P and sliding velocities ν s , taken directly from the SFB. Traces are monitored via bending of the shear springs K s in response to back-and-forth lateral motion Δ x 0 applied to the top surface (for example, top trace in a ), see inset to Fig. 1 . ( a ) Typical traces showing variation of F s with increasing loads F n , corresponding to increasing P , at fixed ν s (200 nm s −1 ). Extraction of signals from noisy profiles is described below ( d ). In other measurements, F s was determined at decreasing F n and P . ( b ) Summary of F s versus F n data from traces such as in a , at ν s =200 nm s −1 . The lines correspond to friction coefficients μ (= F s / F n ) as indicated. Different symbols (coloured to highlight difference) correspond to different contact points, including different experiments. Full symbols: increasing F n ; empty symbols: decreasing F n , and each shape of symbols is for increasing or decreasing load at a given contact point. The lower inset shows typical fringe-tip flattening at high P (enabling checks of the Hertzian expression used to evaluate P , Methods). ( c , d ) Typical F s ( t , ν s ) traces at the high ( F n =6 mN) and low ( F n =0.1 mN) load regimes, respectively, at fixed loads F n , at increasing velocities ν s applied to the top surface. In other measurements, F s was determined at decreasing ν s . For the traces shown, the amplitudes Δ x 0 indicated are fixed, whereas the frequencies vary as shown. Where the signal is comparable with the noise level, as in b , the F s values are extracted at the respective drive frequencies using Fast Fourier Transform of the data to frequency ( ω )-dependent F s ( ω ), as indicated on the right of d . Full size image Sliding velocity dependence of shear forces The variation of shear force F s with sliding velocity ν s , shown in Figs 3 and 4 , exhibits two forms depending on the load regime. For higher loads, the top two data sets in Fig. 3 , where the surface separation is D = D h =0.48±0.16 nm (Methods), the variation is close to logarithmic, F s = A + B .ln( ν s ), where A and B are constants, over some orders of magnitude in ν s . Two typical data sets in the high-load regime are shown in Fig. 3 (black and red squares), and we note also the lower scatter in each arising from the fact that they are at given contact points, and thus at fixed relative orientations of the opposing mica surfaces. In the lower loads regime, lower data set in Fig. 3 and on an expanded scale in Fig. 4 , where D = D l =0.85±0.15 nm (Methods), the variation is much closer to linear, F s – F s,0 = C . ν s , where F s,0 (Methods) and C are independent of ν s . In both regimes F s varies reversibly with the sliding velocity (within the scatter). In Fig. 4 , the range of F s and ν s values earlier studies [3] , [19] is shown in the yellow highlighted rectangle. 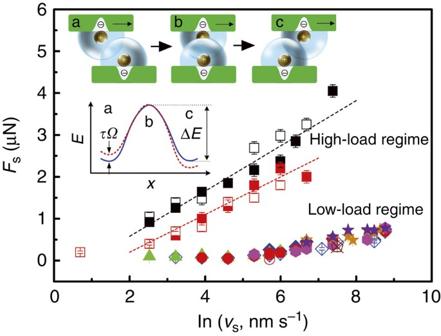Figure 3: Variation of shear forceswith sliding velocity. Variation of shear forceFswith sliding velocityνs, from traces as inFig. 2c,d, in both high- and low-load regimes (plotted asFsversus ln(νs)). Shown are data at two high loads (black squares:Fn=8 mN; red squares:Fn=6 mN) for which the surface separationD=0.48±0.15 nm; and at several low loads (all other symbols, in range aboutFn=0.1–0.2 mN), for whichD=0.85±0.15 nm (for clarity, the orange star data symbols, which haveFs,0values larger by some 0.5 μN than typicalFs,0values (see Methods) have been reduced by this amount). Full and empty symbols are at increasing and decreasingνs, respectively. The variation in the high-load regime, straight broken lines, isFs=A+B.ln(νs), whereAandBare constants. TheFs(νs) variation in the low-load regime is amplified inFig. 4. The inset cartoon illustrates the sliding mechanism for the high-load regime considered in the text and Methods (the cartoon is approximately to scale, indicating the mica surfaces at separationD=0.5 nm, where the negatively charged lattice sites are 0.7 nm apart3,18,20,26, the bare Na+ion diameters are 0.2 nm and the diameter of the first hydration shell about the Na+is ca 0.7 nm (refs23,24,27)). Hydrated ions are localized at the oppositely charged surface sites and need to move past each other as the surfaces slide (a→b→c). As they do so they must overcome an energy barrier ΔEwith a maximum at the point of closest ion–ion approach (b). An applied shear stress τ will modify the energy barrier as indicated by the broken curve (Methods). The error bars represent standard deviations. Figure 3: Variation of shear force s with sliding velocity. Variation of shear force F s with sliding velocity ν s , from traces as in Fig. 2c,d , in both high- and low-load regimes (plotted as F s versus ln( ν s )). Shown are data at two high loads (black squares: F n =8 mN; red squares: F n =6 mN) for which the surface separation D =0.48±0.15 nm; and at several low loads (all other symbols, in range about F n =0.1–0.2 mN), for which D =0.85±0.15 nm (for clarity, the orange star data symbols, which have F s,0 values larger by some 0.5 μN than typical F s,0 values (see Methods) have been reduced by this amount). Full and empty symbols are at increasing and decreasing ν s , respectively. The variation in the high-load regime, straight broken lines, is F s = A + B .ln( ν s ), where A and B are constants. The F s ( ν s ) variation in the low-load regime is amplified in Fig. 4 . The inset cartoon illustrates the sliding mechanism for the high-load regime considered in the text and Methods (the cartoon is approximately to scale, indicating the mica surfaces at separation D =0.5 nm, where the negatively charged lattice sites are 0.7 nm apart [3] , [18] , [20] , [26] , the bare Na + ion diameters are 0.2 nm and the diameter of the first hydration shell about the Na + is ca 0.7 nm (refs 23 , 24 , 27 )). Hydrated ions are localized at the oppositely charged surface sites and need to move past each other as the surfaces slide (a→b→c). As they do so they must overcome an energy barrier Δ E with a maximum at the point of closest ion–ion approach (b). An applied shear stress τ will modify the energy barrier as indicated by the broken curve (Methods). The error bars represent standard deviations. 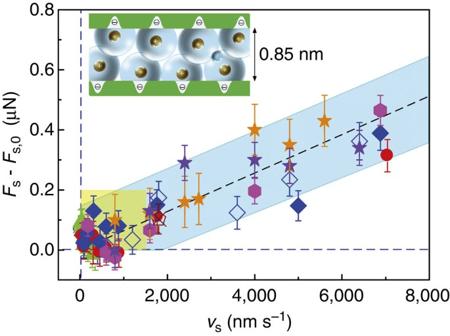Figure 4: Variation of shear forceswith sliding velocity in the low-load regime. Variation of shear force with sliding velocity in the low-load regime, fromFig. 3. The data are plotted as (Fs−Fs,0) versusνs, whereFs,0is a small systematic signal unrelated to the shear force between the surfaces, and is determined separately for each contact point (Methods). Different symbols (coloured to highlight difference) are from different experiments or different contact points within an experiment. Full and empty symbols correspond to increasing and decreasingνs, respectively. From the slope of the blue band an effective viscosity for the confined filmηeff=0.22±0.07 Pa.s is evaluated (see text). The yellow rectangle indicates the range of sliding velocities applied and corresponding shear forces measured for all previous experiments3,19of sliding between mica surfaces across high-salt concentrations, 0.1–0.01 M, of alkali metal ions (in the low-load regime). The inset cartoon is approximately to scale, seeFig. 3caption, forD=0.85 nm, and illustrates the filling by the hydration water of this intersurface gap (see text). The error bars represent standard deviations. Full size image Figure 4: Variation of shear force s with sliding velocity in the low-load regime. Variation of shear force with sliding velocity in the low-load regime, from Fig. 3 . The data are plotted as ( F s − F s,0 ) versus ν s , where F s,0 is a small systematic signal unrelated to the shear force between the surfaces, and is determined separately for each contact point (Methods). Different symbols (coloured to highlight difference) are from different experiments or different contact points within an experiment. Full and empty symbols correspond to increasing and decreasing ν s , respectively. From the slope of the blue band an effective viscosity for the confined film η eff =0.22±0.07 Pa.s is evaluated (see text). The yellow rectangle indicates the range of sliding velocities applied and corresponding shear forces measured for all previous experiments [3] , [19] of sliding between mica surfaces across high-salt concentrations, 0.1–0.01 M, of alkali metal ions (in the low-load regime). The inset cartoon is approximately to scale, see Fig. 3 caption, for D =0.85 nm, and illustrates the filling by the hydration water of this intersurface gap (see text). The error bars represent standard deviations. Full size image Our main findings are that the sliding friction forces vary with sliding velocity either logarithmically or linearly, depending on the surface separation regimes, which in turn depends on the loads (designated high load and low load, respectively). The crucial question is: what are the dominant dissipation modes in these two regimes? The logarithmic variation of the friction with sliding velocity at high loads ( Fig. 3 ) is characteristic of Eyring-like rate-activated processes arising from the overcoming of energy barriers, as seen in a number of solid-friction or boundary lubrication studies [21] , [22] . The surface separation D h =0.48±0.15 nm is comparable with twice the diameter of the bare Na + ions (~0.2 nm each [23] , [24] ) localized at the surface charges. Thus, in this regime, the sliding of the two surfaces may be understood in terms of a process where a potential energy Δ E of sliding surface-localized ions past each other needs to be overcome (Methods), as indicated in the scaled cartoon inset in Fig. 3 . Energy dissipation occurs predominantly when phonons (degraded into heat) are generated in the irreversible conversion of potential to kinetic energy following the overcoming of the energy maximum [25] . Such frictional processes may be described by the following relation, derived for this configuration in the Methods section: Here is the contact area, k B and T are Boltzmann’s constant and the absolute temperature, and Ω is the stress-activated volume associated with sliding of ions past each other; the constant is linear in Δ E . This mechanism also accounts for the relatively large scatter in F s in Fig. 2b : the magnitude of Ω and Δ E and thus of the friction force F s depends on the relative position of the localized counterions on the opposing surfaces sliding past each other. As counterions are localized at the negatively charged lattice sites on the mica surface, the energy barrier to their sliding past each other ( Fig. 3 cartoon) depends on the relative orientation of the opposing lattices. Where the relative orientation is sufficiently unfavourable, this may lead to friction large enough to tear the mica surfaces, as happened in several cases (Methods). This relative offset of the opposing lattices was not controlled in our study, and we attribute the scatter in the F s versus F n plot in Fig. 2b to such differences between different experiments and contact points. We note that the scatter for a given contact point (where the relative orientation and thus Δ E and Ω are expected to be constant (Methods)) is much lower, as expected (see, for example, the two high-load data sets in Fig. 3 ). Although the F s ( ν s ) behaviour in the high-load regime is dominated by dissipation via activated crossing of energy barriers arising from counterion-localization on the confining surfaces, the behaviour in the lower-load regime, D l =0.85±0.15 nm, reveals the dissipation in the sheared hydration shells themselves. This is a far more general effect, relevant whenever contacting hydrated species are in relative motion. The variation F s ( ν s )– F s,0 = C . ν s in this regime, blue band in Fig. 4 , comprises a small systematic component F s,0 arising from indirect coupling of the surfaces to the apparatus (Methods), and a term linearly dependent on the sliding velocity characteristic of viscous dissipation. At the surface separation D l , the number density ρ c/i of counterions trapped between the surfaces is ρ c/i =(2 σ − / D l ), where σ − ≈2 nm −2 is the areal density of ionizable lattice sites on the mica surface, each of which is associated with a trapped, hydrated Na + counterion [3] , [18] , [20] , [26] . This density is determined by the negatively charged sites on the mica, which arise when the K + ions from the mica surface lattice are lost to solution when it is immersed in water. The number of water molecules n w per Na + ion trapped in the gap is then given by n w = ρ H2O / ρ c/i ≈6, where ρ H2O is the number density of water molecules=(density of water)/(mass of a water molecule). Thus, n w is comparable with the number, 4–7, of water molecules in the first (most tightly held) hydration shell of a Na + ion [23] , [27] . This implies that essentially all the water molecules in the gap D l ≈0.85 nm belong to primary hydration shells of the trapped counterions. This observation enables us to evaluate a dissipation characterized by an effective shear viscosity η eff of the hydration shells. Applying a Newtonian relation [28] to the film, the shear stress may be written as , where the shear rate . Thus, (∂ F s /∂ ν s )=( eff / D l ), and from the measured slope C of the blue band in Fig. 4 , we may extract the effective viscosity of the confined film, η eff =0.22±0.07 Pa.s. This value η eff of the hydration shell viscosity is some 250-fold larger than the viscosity of bulk water η H20 =8.8 × 10 −4 Pa.s at 25 °C. We emphasize that the viscosity of water that is not in hydration layers surrounding a charge, but is likewise confined to subnanometre films by mica surfaces, has an effective value that is comparable to η H20 (ref. 29 ) and so is also some two orders of magnitude smaller than η eff . In other words, it is not the subnanometre confinement that leads to the much higher viscous dissipation of the hydration water, but rather its being within the primary hydration shell surrounding the counterion charges. We also confirmed (see Supplementary Fig. 1 and Supplementary Note 1 ) that when lower loads are applied so that the equilibrium separation of the surfaces significantly exceeds the value (ca 0.8 nm) at which the confined water molecules all belong to the hydration shells, the effective viscosity within the gap in the linear regime tends—within the scatter of the data—towards that of bulk water. This measured value of the hydration shell dissipation is consistent with the exchange rate ω H2O,Na+ of water molecules in the hydration shell of Na + with bulk water molecules [23] . The value of ω H2O,Na+ ≈10 9 s −1 corresponds to an exchange time τ H2O,Na+ =(1/ ω H2O,Na+ )≈10 −9 s, which may be taken as approximately the relaxation time of water within the hydration shells. This compares with relaxation times τ H2O ≈10 −11 s in bulk water [28] . On general grounds [30] , one expects liquid viscosity η to be proportional to molecular relaxation times τ , η = Gτ (where G is a limiting high-frequency modulus), as long as the shear rate is much lower than τ −1 , as is the case in the present study. The ratio ( τ H2O,Na+ / τ H2O )≈100 is thus consistent with the ~250-fold enhancement of the hydration shell viscosity η eff relative to η H20 . Molecular dynamics simulations of hydrated K + ions, confined to films of thickness D between mica surfaces [31] , show an approximately two orders of magnitude enhancement of low-shear-rate viscosity (relative to bulk water) at D =0.94 nm, and are thus also consistent with our findings. Also consistent with our findings is an earlier conjecture made in ref. 3 . Likewise, for similarly confined Na + ions where additional dissipation pathways may be active, the lower limit of values measured in ref. 4 , which utilizes a resonance-damping approach, is consistent with our findings for the corresponding surface separation range. Earlier findings on lubricated sliding between hydrated surface layers including hydrated ions [3] , [4] , [5] , surfactants [6] , [7] , [8] , polymers [10] , [11] , [12] or liposomes [9] could not reveal the underlying process. This is because the measured friction was a convolution of the hydration lubrication with other dissipation pathways, such as the activated processes described above, or deformation [6] , [7] , [8] , [9] or entanglement [10] , [11] , [12] effects in the boundary layers themselves. The present study elucidates this—for the simplest case of trapped, hydrated ions—by unravelling this convolution and separating the dissipation modes (and in future work it would be interesting to examine different aspects such as the case of different ions and of the transition between the regimes). In particular, we identify the dissipation pathway and the viscous losses in the bound hydration layers alone, which are characterized by an effective viscosity orders of magnitude larger than that of non-hydration water. This insight largely accounts for the massive friction reduction via the hydration lubrication mechanism recently described in many systems [3] , [5] , [6] , [7] , [8] , [9] , [10] , [11] , and has implications for better design of boundary lubricants and their interfacial vectors in biomedical contexts. Moreover, it provides a framework for understanding lubrication processes in living systems where hydration layers are ubiquitous. Experimental Water used was highly purified (Barnstead NanoPure, resistivity 18.2 MΩ cm, total organic content nominally <1 p.p.b.). Salts, used as received, were 99.99% (Merck) and 99.995% (Fluka). The SFB method is described in detail in ref. 32 . Contact areas A between the surfaces were evaluated using the Hertzian contact mechanics relation r =( F n R / K ) 1/3 for the radius of the flattened circular contact of two crossed cylinders, radius R , under a load F n , where K is an effective mean modulus of the mica/glue layer determined in separate measurements as K =3 × 10 9 N m −2 . The area is then = πr 2 . Comparison of these values with contact areas obtained by directly measuring the flattening of the optical fringe tips (as in Fig. 2b in the main paper) in the high-load regime were generally within 30% of each other over all experiments. Mean pressures were evaluated as P =( F n / A ). At higher loads ( P >ca 1.5 MPa), the mica surfaces often tore on shear, due probably to either trace contamination or, more likely, unfavourable relative orientation of the surfaces (see main text) or a combination of the two, and were aborted following damage. Only experiments where both F n ( D ) and F s profiles were reversible and reproducible (within the scatter) with respect to load and sliding velocities, and thus clearly undamaged, are reported (results are reported from all nine independent experiments in which no damage occurred, that is, different pairs of mica sheets, with different contact points in each; in a substantial number of other experiments, the mica surfaces tore on strong compression and shear, which we attribute to the unfavourable relative orientation of the mica surfaces, see main text and below. In experiments where such damage occurred, no surface interactions could be measured and the experiments were aborted). The weak coupling of the shear springs of the SFB to the body of the apparatus results in a small systematic signal F s,0 at the drive frequency (considered in ref. 29 ), and depends on the amplitude Δ x 0 of lateral motion applied to the top surface (inset to Fig. 1 ). It is evaluated for each run (of different Δ x 0 ) from measurements at large D where the shear force between the surfaces vanishes. The D h and D l values are the mean of 23 and 25 measurements in the high-load (ca 5–8 mN) and low-load (ca 0.1–0.2 mN) regimes respectively, where the quoted uncertainty is twice the standard error in the mean given by Peter’s formula [33] . Rate activated sliding The logarithmic variation of F s with ν s in equation 1 of the main text is similar to analogous relations for sliding but adhering surfaces [21] , [22] . Here we sketch a derivation for the configuration inset to Fig. 3 , based on a simplified treatment of the Eyring theory of liquid viscosity [28] . In the unperturbed system (no shear stress), the frequency ν 0 at which a localized ion can overcome the potential barrier Δ E to crossing to an adjacent energy minimum is ν 0 = ν c .exp(−Δ E /k B T ), where ν c is a characteristic frequency. If a shear stress τ acting on the localized ions is applied to the right, say, the potential is modified by τ Ω as indicated by the broken curve in the inset to Fig. 3 , where Ω is an effective stress-activated volume. The net rate ν of jumping to the right then becomes where Ω, the effective stress-activated volume, may be much larger than an ionic volume. As long as τ Ω ≫ k B T , we may ignore exp(– τ Ω/ k B T ) relative to exp( τ Ω/ k B T ) in (equation 2), giving The sliding velocity ν s is related to the net jump frequency ν , as ν s = νd , where d is the mean amplitude of a jump. Substituting for ν =( ν s / d ) and taking logarithms of both sides, we have finally giving equation 1 in the text (we note that the constant is linear in Δ E ) From the slope ∂ F s /∂(ln( ν s ))≈0.5 × 10 −6 N in Fig. 4 , we extract a value for Ω≈2 × 10 −23 m 3 . We can check that indeed τ Ω≈3 × 10 −20 J>> k B T (≈4 × 10 −21 J), which is the assumption underlying in equation 3. How to cite this article : Ma, L. et al. Origins of hydration lubrication. Nat. Commun. 6:6060 doi: 10.1038/ncomms7060 (2015).